Carbon nanotube–liposome supramolecular nanotrains for intelligent molecular-transport systems Biological network systems, such as inter- and intra-cellular signalling systems, are handled in a sophisticated manner by the transport of molecular information. Over the past few decades, there has been a growing interest in the development of synthetic molecular-transport systems. However, several key technologies have not been sufficiently realized to achieve optimum performance of transportation methods. Here we show that a new type of supramolecular system comprising of carbon nanotubes and liposomes enables the directional transport and controlled release of carrier molecules, and allows an enzymatic reaction at a desired area. The study highlights important progress that has been made towards the development of biomimetic molecular-transport systems and various lab-on-a-chip applications, such as medical diagnosis, sensors, bionic computers and artificial biological networks. Human activities (for example, thought, emotion and behaviour) are directly formed by biological network systems. Biological network systems such as inter/intra-cell-signalling systems are handled in a sophisticated manner by the molecular transport of molecular information (low-molecular-weight compounds, proteins and genes and so on) [1] . Over the past few decades, there has been a strong interest in the development of molecular-transport systems using microorganisms [2] , naturally occurring biomolecular motors [3] , [4] and synthetic micro-nanoscale robots (micro-nanobots) [5] , [6] , [7] , [8] . However, the following key technologies are not sufficiently developed to realize optimum performance from the transportation method: directional propagation of transporters [4] , [9] , [10] , [11] , controlled release [8] of carrier molecules and transmission/reception systems (artificial molecular signalling; expression of significant biochemical reactions in the targeted sites) for transferred carrier molecules [3] , [6] . Nanomaterials are potentially promising for a number of scientific and technological applications [12] . For the creation of functional nanomaterials for various nanobiosystems, molecular self-assembly technologies have attracted significant attention, as they are easily processed [12] . In particular, liposomes are one of the most well-known self-assembled materials and have numerous uses as biochemical and biophysical tools because of their many attractive properties, which includes encapsulating a variety of molecules (drugs, peptides, proteins and genes and so on) and exhibiting dramatic conformation changes due to external physical or chemical stimulations (pH, light and temperatureand so on) [13] , [14] , [15] , [16] . On the other hand, carbon nanotubes (CNTs) offer a unique combination of electrical, mechanical, thermal and optical properties that make them highly promising materials for numerous applications [17] , [18] , [19] , [20] , [21] , [22] , [23] , [24] . We have been investigating the use of laser-induced CNTs as a potent photothermal nanomaterial in various thermal applications [17] , [18] , [19] , [20] , [21] , [22] , [23] , [24] . Of several photothermally active nanomaterials that were considered, CNTs are particularly interesting because of the extraordinarily high efficiency of their photothermal energy conversion and high light-absorption cross-section over a wide range of wavelengths [17] , [18] , [19] , [20] , [21] , [22] , [23] , [24] . The functionalization of CNTs is the next key step for the integration of these new materials into different systems for technological and biomedical applications [25] . In this study, we demonstrate that (1) an electrical train-like nanobot based on a CNT and temperature-responsive liposome (CNT–liposome nanotrain) can be formed by a self-assembly technology; (2) the CNT–liposome nanotrains successfully function in microdevices for various applications, such as the solving of mazes and molecular transportations after the application of voltage and because of the photothermal property of CNT; and (3) the electric- and light-driven CNT–liposome nanotrains effectively illustrated the enzymatic reaction at the targeted position. Our newly developed molecular-transport system, which is based on the photoinduced-CNT–liposome nanotrains, can easily trigger the unloading of molecules and an enzymatic reaction in a targeted area in a non-contact manner. This is performed using a highly focused external laser beam. Our designed supramolecular nanotrains and the intelligent molecular-transport system provide a starting point for the exploration of more sophisticated biomimetic molecular-transport systems with directionally controlled motion, on-time controlled release of carrier molecules and various biochemical reactions derived from the receipt of functional molecules at the desired area. Characterization of nanotrains To develop an intelligent molecular-transport system, we synthesized the CNT–liposome nanotrains using a self-assembly technology ( Fig. 1 ) (see Methods for details). However, generally, CNTs are not dispersed in solvents because of their strong tendency to aggregate [17] , [18] , [19] , [20] , [21] , [22] , [23] , [24] . Hence, we employed a highly water-dispersible avidin–polyethylene glycol-2,000 (PEG 2,000 , molecular weight of PEG=2,000)–phospholipid (PL)-functionalized-single-walled CNT (SWNT) (avidin–PEG 2,000 –PL–SWNT) complex by the non-covalent approach [17] , [18] , [19] , [20] , [21] , [22] , [23] , [24] ( Fig. 1a ). The hydrocarbon chains of PLs were adsorbed onto the graphitic surfaces of SWNTs via van der Waals and hydrophobic interactions, whereas the hydrophilic PEG chains extended into the aqueous phase to impart solubility [23] . On the other hand, generally, the functional liposomes were prepared by labelling 1,2-distearoyl-sn-glycero-3-phosphoethanolamine- N -[biotinyl(polyethyleneglycol)-2,000] (biotin–PEG 2,000 –PL) and N -(7-nitrobenz-2-oxa-1,3-diazol-4-yl)dioleoyl phosphatidylethanolamine (NBD–PE) molecules on the surface of liposomes. In addition, the functional liposomes are composed of dipalmitoylphosphatidylcholine, hydrogenated soybean phosphatidylcholine (HSPC) and cholesterol (see Methods for details). Furthermore, the functional liposomes spontaneously bind to SWNTs through the ligand–receptor interaction of biotin–avidin, and NBD molecules [15] on the liposomes enable the tracking of the CNT–liposome nanotrain movement in the microdevices as a fluorescent tracer. Fluorescence microscopy analysis showed that the Brownian motion of green fluorescent CNT–liposome nanotrains (average size ≤1 μm) is observed in aqueous solution ( Fig. 1b ). 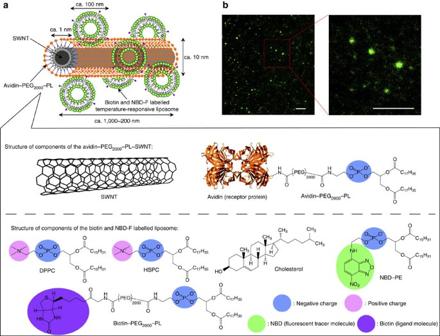Figure 1: Structural characterization of CNT–liposome nanotrains. (a) Schematic illustration of the CNT–liposome nanotrain. (b) Fluorescence microscopic images of CNT–liposome nanotrains. Magnification: X100. Scale bars, 10 μm. These visible green fluorescent nanotrain particles are observed only when the SWNT and liposome are mixed in a predetermined stoichiometry ( Table 1 and Fig. 2 ). We investigated the compounding ratio of SWNTs and liposome for the synthesis of microscopically detectable fluorescent nanotrains. Visible green fluorescent particles are observed only when the SWNT and liposome are mixed in a specific compounding ratio ( Table 1 ; entry 1) ( Fig. 2a ). As a result, the entry 1 sample shows the maximum fluorescence intensity. On the other hand, visible black aggregations resulting from CNTs are formed in the cuvette in cases where there is a low liposome-compounding ratio ( Table 1 ; entry 2 and 3). This is believed to be caused by the precipitation of CNTs when a small amount of liposomes form tightly roped bundles via the avidin–biotin interaction ( Fig. 2b ). Although the background fluorescence intensity is relatively high, visible fluorescent particles are not observed in the case of a high liposome-compounding ratio ( Table 1 ; entry 4), because of the low synthetic yield of nanotrains ( Fig. 2d ). We can detect neither the avidin–PEG 2,000 –PL–SWNT nor the functional liposome by fluorescence microscopy because of the detection limitations of microscopy ( Table 1 ; entries 5 and 6) ( Fig. 2e ). Also, a mixed solution of the functional liposome and NH 2 –PEG 2,000 –PL–SWNT does not exhibit fluorescence because of incomplete supramolecular complexes ( Table 1 ; entry 7) ( Fig. 2g ). These results clearly indicate that the optimum concentrations of the avidin–PEG 2,000 –PL–SWNT and the functional liposome are ~5 and 20,000 nM, respectively. Next, the CNT–liposome nanotrain was structurally characterized by transmission electron microscopy (TEM) ( Fig. 3 ). TEM analysis of the CNT–liposome nanotrain revealed that spherical liposomes (average diameter≈100 nm) are attached on the surface of an avidin–PEG 2,000 –PL–SWNT nanofibre (average diameter≈10 nm, length≈200–1,000 nm), as shown in Fig. 1a . We also observed that the lipid-coated fibreform SWNTs became entangled on the surface of liposomes and resulted in the formation of aciniform structures. These results clearly show that the synthesized CNT–liposome nanotrains have supramolecular nanostructures, and their luminary fluorescence facilitates the observation of microscopic fluorescence. Figure 1: Structural characterization of CNT–liposome nanotrains. ( a ) Schematic illustration of the CNT–liposome nanotrain. ( b ) Fluorescence microscopic images of CNT–liposome nanotrains. Magnification: X100. Scale bars, 10 μm. Full size image Table 1 Synthesis of CNT–liposome nanotrain. 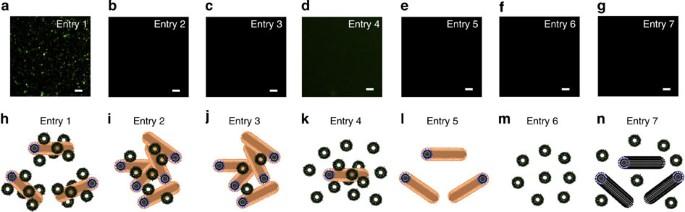Figure 2: Effect of SWNT and liposome concentrations on the nanostructure of CNT–liposome nanotrains. (a–g) Fluorescence micrographs of various CNT–liposome nanotrains inTable 1(entry 1–7). Scale bars, 10 μm. (h–n) Schematic illustrations of various CNT–liposome nanotrains inTable 1(entry 1–7). Visible green fluorescent nanotrain particles are observed only when the SWNT and liposome are mixed in a specific compounding ratio (entry 1 inTable 1). Graphics depict the expected nanotrain conformations (Fig. 2h–n). These results clearly indicate that the optimum compounding ratio of the avidin–PEG2,000–PL–SWNT and functional liposome is 1:4,000 for further experiments (entry 1 inTable 1). Full size table Figure 2: Effect of SWNT and liposome concentrations on the nanostructure of CNT–liposome nanotrains. ( a – g ) Fluorescence micrographs of various CNT–liposome nanotrains in Table 1 (entry 1–7). Scale bars, 10 μm. ( h – n ) Schematic illustrations of various CNT–liposome nanotrains in Table 1 (entry 1–7). Visible green fluorescent nanotrain particles are observed only when the SWNT and liposome are mixed in a specific compounding ratio (entry 1 in Table 1 ). Graphics depict the expected nanotrain conformations ( Fig. 2h–n ). These results clearly indicate that the optimum compounding ratio of the avidin–PEG 2,000 –PL–SWNT and functional liposome is 1:4,000 for further experiments (entry 1 in Table 1 ). 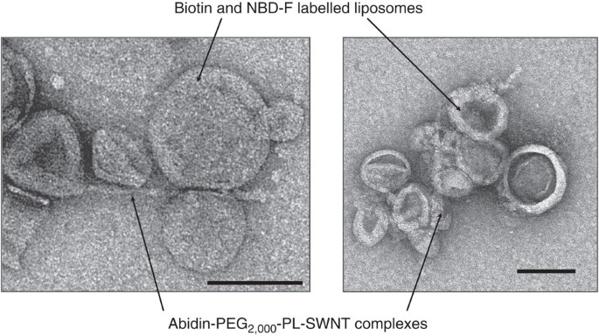Figure 3: TEM images of CNT–liposome nanotrains. Sample concentration for these observations: SWNT=5 nM, liposome=20,000 nM. Scale bars, 100 nm. Full size image Figure 3: TEM images of CNT–liposome nanotrains. Sample concentration for these observations: SWNT=5 nM, liposome=20,000 nM. Scale bars, 100 nm. Full size image Nanotrains movement in the microdevice The ability to use electrical control for the direction and motion of CNT–liposome nanotrains in a microdevice is illustrated in Fig. 4 . First, we prepared a polydimethylsiloxane (PDMS) microdevice based on a straight microchannel (width: 100 μm, depth: 50 μm) to investigate the microscale behaviour of CNT–liposome nanotrains by applying a voltage ( Fig. 4a ). To prevent the adhesion of nanotrains to the surface of the microchannels, the fabricated microdevice was treated with a hydrophilic polymer (Methods). In addition, 20 wt% of dextran was introduced into the microchannel to prevent the undesired permission of nanotrains to enter a microchannel caused by molecular diffusion (Methods). The synthesized CNT–liposome nanotrains are negatively charged in the 4-(2-hydroxyethyl)-1-piperazineethanesulfonic acid (HEPES) buffer (pH 7.1) (zeta potential=−0.21±1.6 mV). In this way, the CNT–liposome nanotrains can move to the positively charged goal position from the negatively charged start position by the application of voltage. Green fluorescent CNT–liposome nanotrains gradually move straight ahead to the goal position after a voltage is applied (50 V), as indicated by fluorescence microscopy ( Fig. 4c and Supplementary Movie 1 ). Figure 2d shows the absolute and relative speeds of the CNT–liposome nanotrains in a microchannel with the application of different voltages and current outputs. Under these conditions, the nanotrains can reach absolute speeds of ~700 μm s −1 , which correspond to a relative speed of ~1,200 body lengths (bl) per second. Thus, we report the realization of fast, electric-driven nanobots with speeds that are comparable to that of catalytic self-propelled microengines (ca. 200 bl s −1 ) [5] and some bacteria (ca. 50–150 bl s −1 ) [5] . Figure 2e reveals the fluorescence intensity curves for the moved CNT–liposome nanotrains with the application of various voltages (50–400 W). We found that there was a significant increase in the fluorescence intensity of nanotrains as the voltage output increased. On the other hand, it is well known that the electrocataphoresis of DNA in a micro-nanodevice is rapid because of the small cavity in micro-nanochannels [26] . Hence, the speed of the CNT–liposome nanotrain was investigated for comparison with that of the representative DNA molecule (λ phage DNA), which has a negative charge that is derived from phosphate backbone (zeta potential=−16.3±0.82 mV) ( Fig. 4f ). In the present system, the average speed of the CNT–liposome nanotrains is approximately two times higher than that of λ phage DNA molecules. This may be due to the physical migration barrier of molecules in the dextran gel construct ( Fig. 4g ). From fluorescence microscopy, the particle sizes of the λ phage DNA molecules intercalated with GelRed (average size≈10 μm) are obviously greater than those of CNT–liposome nanotrains (average size≤1 μm) ( Fig. 4h and Supplementary Movie 2 ). Furthermore, to realize the advanced electronic regulation of nanotrains, we investigated the switchback control of the CNT–liposome nanotrain movements in a microchannel ( Fig. 4i ). The direction of the nanotrain’s movement is easily controlled using this mechanical switchback feature in a manner similar to that of an electric train ( Fig. 4j and Supplementary Movie 3 ). These results completely indicate that electric-driven CNT–liposome nanotrains can be directionally moved in a microdevice similar to ‘electrotaxis’, which is the movement of organisms towards or away from a source of electrostimulation using a biased-random-walk process [27] . 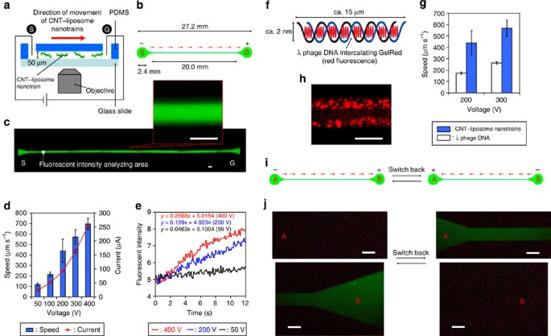Figure 4: Electrical control of CNT–liposome nanotrain movement. (a) Schematic illustration of the experiment system. S, start; G, goal. (b) Design drawing of the microdevice based on a straight microchannel. Red arrows show the direction of CNT–liposome nanotrain movement. (c) Movement of the CNT–liposome nanotrains in a straight microchannel after applying a voltage. The white square shows the location at which the fluorescence intensity of the moving CNT–liposome nanotrains was analysed. Applying a voltage=50 V. Magnification of the inset close-up figure: X10. Scale bars, 100 μm. (d) Speed of the CNT–liposome nanotrains and current in microchannel versus applying a voltage. (e) Fluorescent intensity curves of the moved CNT–liposome nanotrain at various applied voltages (50–400 W). (f) Schematic illustration of the single λ phage DNA intercalated with GelRed molecules. (g) Fluorescence microscopic image of the λ phage DNA molecules in a straight microchannel. Applying a voltage=200 V. Magnification: X10. (h) Speed of the CNT–liposome nanotrains and λ phage DNA molecules in a straight microchannel after applying voltage. Scale bar, 100 μm. (i) Switchback control of the CNT–liposome nanotrain movement. Red arrows show the direction of CNT–liposome nanotrain movement. (j) A direct observation of the switchback movement of the CNT–liposome nanotrains by fluorescence microscopy. Magnification: X10. Applying voltage=300 V. Scale bars, 100 μm. Figure 4: Electrical control of CNT–liposome nanotrain movement. ( a ) Schematic illustration of the experiment system. S, start; G, goal. ( b ) Design drawing of the microdevice based on a straight microchannel. Red arrows show the direction of CNT–liposome nanotrain movement. ( c ) Movement of the CNT–liposome nanotrains in a straight microchannel after applying a voltage. The white square shows the location at which the fluorescence intensity of the moving CNT–liposome nanotrains was analysed. Applying a voltage=50 V. Magnification of the inset close-up figure: X10. Scale bars, 100 μm. ( d ) Speed of the CNT–liposome nanotrains and current in microchannel versus applying a voltage. ( e ) Fluorescent intensity curves of the moved CNT–liposome nanotrain at various applied voltages (50–400 W). ( f ) Schematic illustration of the single λ phage DNA intercalated with GelRed molecules. ( g ) Fluorescence microscopic image of the λ phage DNA molecules in a straight microchannel. Applying a voltage=200 V. Magnification: X10. ( h ) Speed of the CNT–liposome nanotrains and λ phage DNA molecules in a straight microchannel after applying voltage. Scale bar, 100 μm. ( i ) Switchback control of the CNT–liposome nanotrain movement. Red arrows show the direction of CNT–liposome nanotrain movement. ( j ) A direct observation of the switchback movement of the CNT–liposome nanotrains by fluorescence microscopy. Magnification: X10. Applying voltage=300 V. Scale bars, 100 μm. Full size image Navigation system Next, we investigated about a higher level of motion control of CNT–liposome nanotrains ( Fig. 5 ). The solving of maze problems is relevant to the everyday issues of urban transportation and experimental psychology and is also one of the model problems in network and graph theory and robotics [28] , [29] , [30] , [31] , [32] . In this study, we posed several problems: finding the shortest paths in the bifurcated microchannel ( Fig. 5a ), the simple maze ( Fig. 5b and Supplementary Fig. S1 ) and the complicated maze ( Fig. 5e ) using biomimetic CNT–liposome nanotrain electrotaxis. These devices have 100-μm-wide and 50-μm-deep microchannels (see Methods). Once in the maze, the CNT–liposome nanotrains move towards the goal position; that is, towards the source of the electrical potential gradient. In doing so, the shortest path was always found through the bifurcated microchannels ( Fig. 5c and Supplementary Movie 4 ). 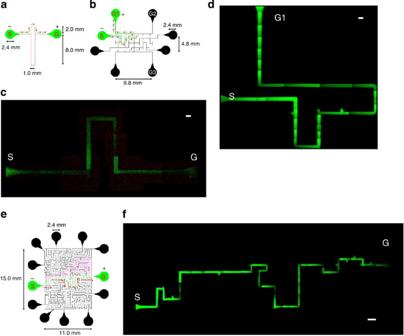Figure 5: Navigations by CNT–liposome nanotrains. (a,b,e) Design drawings of the microdevices based on bifurcated, simple-maze and complicated-maze microchannels, respectively. Red arrows show the direction of CNT–liposome nanotrain movement. Green and pink lines indicate the shortest and the longest paths, respectively. S, start; G, goal; G1, goal 1; G2, goal 2; G3, goal 3. (c) A direct observation of the nanotrain’s behaviour in the bifurcated microchannel after applying a voltage (300 V). Image of the nanotrain movement showing the shortest path between S and G. Scale bar, 100 μm. (d) A direct observation of the nanotrain behaviour in the simple-maze microchannel after applying a voltage (300 V). Image of the nanotrain movement showing the route for the shortest path in the maze. Scale bar, 100 μm. (f) A direct observation of the nanotrain behaviour in the complicated-maze microchannel after applying voltage (300 V). Image of the nanotrain movement showing the quickest route from S to G for a more complex maze. Scale bar, 500 μm. The speed v of the CNT–liposome nanotrains in the microchannel is given by the following equation [33] : Figure 5: Navigations by CNT–liposome nanotrains. ( a , b , e ) Design drawings of the microdevices based on bifurcated, simple-maze and complicated-maze microchannels, respectively. Red arrows show the direction of CNT–liposome nanotrain movement. Green and pink lines indicate the shortest and the longest paths, respectively. S, start; G, goal; G1, goal 1; G2, goal 2; G3, goal 3. ( c ) A direct observation of the nanotrain’s behaviour in the bifurcated microchannel after applying a voltage (300 V). Image of the nanotrain movement showing the shortest path between S and G. Scale bar, 100 μm. ( d ) A direct observation of the nanotrain behaviour in the simple-maze microchannel after applying a voltage (300 V). Image of the nanotrain movement showing the route for the shortest path in the maze. Scale bar, 100 μm. ( f ) A direct observation of the nanotrain behaviour in the complicated-maze microchannel after applying voltage (300 V). Image of the nanotrain movement showing the quickest route from S to G for a more complex maze. Scale bar, 500 μm. Full size image where μ is the mobility of the nanotrains, E is the electric field strength, V is the applied voltage and L the length of the microchannel. Thus, CNT–liposome nanotrains go the shortest path because v is indirectly proportional to L . CNT–liposome nanotrains can be quickly moved to the various targeted goals (G1–G3) from the start by alteration of the electrode position in the goal ( Fig. 5d ; Supplementary Movie 5 and Supplementary Fig. S1 ). Surprisingly, CNT–liposome nanotrains are also able to solve the complicated maze and migrate smoothly along the shortest path within ~1.5 min without ‘steepness’ or ‘errors’ ( Fig. 5f and Supplementary Movie 6 ). These results clearly demonstrate that CNT–liposome nanotrains have intelligent performance navigation for solving mazes using an electrical potential gradient. Molecular-transport system One of the main goals of this study is to demonstrate for the first time the controlled (triggered) release of substrates from CNT–liposome nanotrains ( Fig. 6 ). To accomplish the challenging goal of the controlled release from synthetic CNT–liposome nanotrains, we functionalized the surface of the CNT–liposome nanotrains with a mixed-binding lissamine rhodamine B–sulfonyl phosphatidylethanolamine (Rh–PE) as a temperature indicator [18] , [19] , [20] , [21] and encapsulated calcein as a transporting model molecule into the liposomes ( Fig. 6a ). The present functional liposome has a temperature-responsive property that is designed to structurally destruct at a temperature of greater than 42 °C by adjusting these chemical components [13] , [14] . Recently, we have demonstrated that photoinduced CNTs can operate as exothermic nanomaterials [17] , [18] , [19] , [20] , [21] , [22] , [23] , [24] . Therefore, laser-induced-CNT–liposome nanotrains can trigger the release of calceins from within the liposomes, as shown in Fig. 6a . When the moving CNT–liposome nanotrain in the microchannel was irradiated by a near-infrared (NIR) laser (wavelength: 1,064 nm, laser power: 700 mW (ca. 69 mW μm −2 ), laser spot diameter: ca. 3.6 μm), we immediately observed the shiny green fluorescence caused by released calcein molecules ( Fig. 6d and Supplementary Movie 7 ). The fluorescence of calcein is not observed before laser irradiation because calcein molecules inside the liposomes are self quenched at high concentrations [16] . The controlled release of calceins from the CNT–liposome nanotrains was achieved by the sequential ‘on’ and ‘off’ switching of the NIR laser. 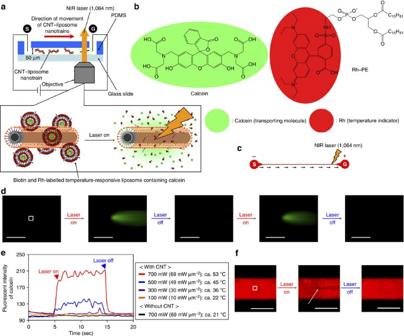Figure 6: Molecular-transport system by CNT–liposome nanotrains. (a) Concept of molecular transportation by CNT–liposome nanotrains. (b) Chemical structure of calcein and Rh–PE. (c) Design drawing of the microdevice based on a straight microchannel for molecular transportation. Black arrows show the direction of CNT–liposome nanotrain movement. S, start; G, goal. (d) Sequential calcein release by laser-induced-CNT–liposome nanotrains. The white dot square shows the location at which the fluorescence intensity of released calcein molecules was analysed. Magnification: X20. Applying voltage=100 V. Scale bars, 100 μm. (e) Fluorescence intensities of the released calcein molecules at various laser powers (100–700 mW (10–69 mW μm−2)). (f) A direct observation of ultrafast temperature change in the microchannel. The white dot square indicates the location at which the temperature was analysed inFig. 4e. The white arrow indicates the fluorescence quenching of Rh by the photothermal property of CNTs. Magnification: X20. Laser power: 700 mW (69 mW μm−2). Applying voltage=100 V. Scale bars, 100 μm. Figure 6e shows the fluorescence profiles at four different laser powers (100, 300, 500 and 700 mW (10, 30, 49 and 69 mW μm −2 , respectively)). We found that the fluorescence intensity increases significantly with the NIR laser power. Upon laser NIR irradiation, we estimated the temperature of nanotrains utilizing Rh molecules on the liposomes ( Fig. 6f and Supplementary Movie 8 ). The fluorescence quenching of Rh for the nanotrains in the microchannel was observed almost immediately (below 0.03 s) upon NIR laser irradiation and is similar to our previous studies [18] , [19] , [20] , [21] . In addition, the temperatures at laser powers of 100, 300, 500 and 700 mW (10, 30, 49 and 69 mW μm −2 , respectively) increased from 21 °C to 22, 36, 45 and 53 °C, respectively ( Fig. 6e ). There were no fluorescent changes illustrating the release of calcein or changes in temperature during the control experiments without CNTs (only functional liposome). Figure 6: Molecular-transport system by CNT–liposome nanotrains. ( a ) Concept of molecular transportation by CNT–liposome nanotrains. ( b ) Chemical structure of calcein and Rh–PE. ( c ) Design drawing of the microdevice based on a straight microchannel for molecular transportation. Black arrows show the direction of CNT–liposome nanotrain movement. S, start; G, goal. ( d ) Sequential calcein release by laser-induced-CNT–liposome nanotrains. The white dot square shows the location at which the fluorescence intensity of released calcein molecules was analysed. Magnification: X20. Applying voltage=100 V. Scale bars, 100 μm. ( e ) Fluorescence intensities of the released calcein molecules at various laser powers (100–700 mW (10–69 mW μm −2 )). ( f ) A direct observation of ultrafast temperature change in the microchannel. The white dot square indicates the location at which the temperature was analysed in Fig. 4e . The white arrow indicates the fluorescence quenching of Rh by the photothermal property of CNTs. Magnification: X20. Laser power: 700 mW (69 mW μm −2 ). Applying voltage=100 V. Scale bars, 100 μm. Full size image Artificial molecular signalling Molecular transportation is inspired by the observation that communication in biological systems, such as inter/intra-cell signalling, is done through molecules [1] . To construct these biomimetic molecular-transport systems, the most important research challenges are directional propagation, the controlled release of carrier molecules and transmission/reception systems for carrier molecules. As a result, we investigated a transmission/reception system—‘artificial molecular signalling’—in which the enzymatic reaction was triggered by the laser-induced-CNT–liposome nanotrains at the targeted position ( Fig. 7 ). The concept of this artificial molecular signalling is illustrated in Fig. 7a . First, the CNT–liposome nanotrains encapsulating fluorescein digalactoside (FDG) that act as transporters of signal molecules are transferred to the targeted goal reservoir (site G) from the start position (site S) by the application of voltage. Next, directionally migrated CNT–liposome nanotrains in site G are irradiated by an NIR laser (1,064 nm), and FDG molecules are released at the targeted area. It is well known that FDG is a fluorogeneic substrate for β-galactosidase [34] . Hence, non-fluorescent FDG is sequentially hydrolysed by the enzymes in site G, and it then transformed to highly fluorescent fluorescein [34] . We can observe bright-green-coloured fluorescence in site G that is caused by the enzymatic reaction as soon as 700-mW (69 mW μm −1 ) NIR irradiation begins ( Fig. 7b and Supplementary Movie 9 ). There were no changes in the fluorescent observations of the enzymatic reaction when the control experiments without CNTs (only functional liposome) were performed. We conclude that the laser-induced-CNT–liposome nanotrains permit the controlled release of substances and the triggered enzymatic reaction through the molecular-transport system, based on the nanotrain’s electrotaxis and the powerful photothermal property of CNT nanoheaters. 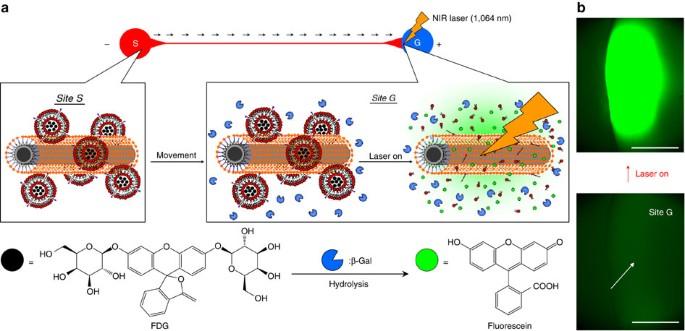Figure 7: Artificial molecular signalling by CNT–liposome nanotrains. (a) Concept of artificial molecular signalling. Black arrows show the direction of CNT–liposome nanotrain movement. (b) Direct observation of enzymatic reaction triggered by artificial molecular signalling. The white arrow indicates the irradiation position of the laser beam. Magnification: X20. Laser power: 700 mW (69 mW μm−2). Applying voltage=100 V. Scale bars, 200 μm. Figure 7: Artificial molecular signalling by CNT–liposome nanotrains. ( a ) Concept of artificial molecular signalling. Black arrows show the direction of CNT–liposome nanotrain movement. ( b ) Direct observation of enzymatic reaction triggered by artificial molecular signalling. The white arrow indicates the irradiation position of the laser beam. Magnification: X20. Laser power: 700 mW (69 mW μm −2 ). Applying voltage=100 V. Scale bars, 200 μm. Full size image We successfully developed a novel supramolecular nanotrain based on CNTs and liposome using the self-assembly technique. The nanotrain enables both directional migration and the solving of mazes in an electric field. In addition, the controlled release of substrates and a triggered enzymatic reaction were successfully achieved at a targeted position using laser irradiation. This study represents an important advance in the creation of programmable and adaptable nanobiosystems. The application of micro-nanobots in micro-nanofabricated environments is an exciting development [2] , [3] , [4] , [5] , [6] , [7] , [8] , [9] , [10] , [11] . Our technology is also going to offer novel possibilities for future developments in lab-on-a-chip applications, such as medical diagnosis, sensors, bionic computers and artificial biological networks. In particular, our system will provide a simulation tool for potential in vivo medical applications, such as remote controlling of untethered micro-nanobots in blood vessels. We believe that these kinds of simulation are very useful for development of advanced drug-delivery systems and nano-surgery of biological system by the use of micro-nanobots. Synthesis of CNT–liposome nanotrains The avidin–PEG 2,000 –PL–SWNT was synthesized as follows. SWNT (2.5 mg) (high-pressure carbon monoxide, super-purified SWNTs (purity>95%); Unidym) and 3-( N -succinimidylocyglutaryl) aminopropyl, polyethyleneglycol carbamyl distearoylphosphatidylethanolamine (NHS–PEG2,000–PL) (5 mg) (molecular weight of PEG chain=2,000; NOF) were sonicated for 15 min in PBS buffer (pH 7.3) (5 ml) on ice (<8 °C) in an ultrasonication bath (USD-2R; AS ONE) to obtain a uniform dispersion. The NHS–PEG 2,000 –PL–SWNT solutions were centrifuged (10,000 g , 15 min, 4 °C) (3500; Kubota). The supernatant was carefully collected after centrifugation. The superfluous NHS–PEG 2,000 –PL was filtered though a polytetrafluoroethylene membrane (pore size=100 nm; Millipore) washed with PBS buffer (50 ml). The black-coloured NHS–PEG 2,000 –PL–SWNT sheet on a polytetrafluoroethylene membrane was dispersed in PBS buffer (5 ml) by sonication for a few minutes. Avidin (1 mg) (Wako) was dispersed in a NHS–PEG 2,000 –PL–SWNT solution (5 ml). After the mixture was vigorously stirred for 3 h at room temperature, it was filtered to remove the unreacted avidin and washed with HEPES buffer (pH 7.1) (50 ml). The obtained avidin–PEG 2,000 –PL–SWNT sheet was dispersed in the HEPES buffer (5 ml) by sonication. The quantity of SWNTs dispersed in the HEPES buffer by avidin–PEG 2,000 –PL molecules was determined through weight measurements by the thorough washing and removal of avidin–PEG 2,000 –PL and was found to be ca. 200 μg SWNT per ml HEPES buffer (ca. 1 μM). The amino-terminated–PEG 2,000 –PL-functionalized SWNT (NH 2 –PEG 2,000 –PL–SWNT) was synthesized in the same way as the avidin–PEG 2,000 –PL–SWNT, with the exception of the functionalization of avidin, except for the process by which avidin is modified. The functional liposomes were synthesized as follows. A mixture of dipalmitoylphosphatidylcholine (Sigma), HSPC (NOF), cholesterol (Sigma), biotin–PEG2,000–PL (molecular weight of PEG chain=2,000; Avanti Polar Lipids) and Rh–PE (Avanti Polar Lipids) or NBD–PE (Avanti Polar Lipids) in the molar ratio of 58.2:29.1:11.6:0.5:0.6 was dissolved in chloroform, and the solvent was removed by evaporation to afford a thin mixed-lipid membrane. The HSPC was generously donated by NOF (Tokyo, Japan). The obtained membrane was further dried under vacuum conditions and dispersed in a 20 mM HEPES-buffered solution containing 150 mM NaCl (pH 7.4) (HBS) by 10 min sonication using a bath-type sonicator at ~65 °C. The obtained liposome suspension was extruded through a polycarbonate membrane (pore size=100 nm; Advantec). The lipid concentration was determined by the choline oxidase method (Phospholipid C Test Wako; Wako). For the loading of calcein (Wako) or FDG (Molecular Probes), a 63-mM calcein solution (pH 7.4) or HBS containing FDG (1 mg ml −1 ) was used for the hydration of the lipid membrane. The free calcein or FDG from the liposome suspension was removed using a Sepharose 4B column (GE Healthcare) with HBS. Finally, the CNT–liposome nanotrains were synthesized by mixing the avidin–PEG 2,000 –DSPE–SWNT with the functional liposomes. The compounding ratio of the SWNT and liposome is 1:4,000 ( Table 1 ). Characterization of CNT–liposome nanotrains The CNT–liposome nanotrains were characterized using a fluorescence microscope (IX71; Olympus) equipped with an electron-multiplying charge-coupled device (EM-CCD) camera (PhotonMAX: 1024B; Princeton Instruments), a TEM (Tecnai G2F20; FEI) (acceleration voltage: 120 kV) and a zeta potential analyser (Nicomp 380 ZLS dynamic light-scattering instrument; Particle Sizing Systems). The TEM observations were supported by the IBEC Innovation Platform, AIST. Before the TEM observation, the CNT–liposome nanotrain in the PBS buffer (pH 7.3) was deposited on a carbon-coated support and negatively stained using a 1% uranyl acetate solution. Microdevices The four varieties of microdevices were based on straight, bifurcated, simple-maze and complicated-maze microchannels (width: 100 μm, depth: 50 μm) and fabricated by soft lithography and photolithography methods. First, the PDMS (Sylgard 184; Dow Corning) base and crosslinker (Sylgard 184; Dow Corning) were mixed at a weight ratio of 10:1, as specified by the manufacturer. Second, the mixture was subjected to shear mixing to ensure the uniform blending of the host matrix and the crosslinker. Next, the mixture was degassed in vacuum. A master was prepared by exposing and developing a photoresist pattern on a silicon wafer (SU-8 50; MicroChem). The PDMS/crosslinker mixture was poured onto the master. After curing, the PDMS substrate was peeled away from the master. Then, the PDMS sheet was punched with holes (diameter: 3 mm) to produce reservoirs. The PDMS and glass (Matsunami) substrates were closely bonded to each other by plasma treatment using a vacuum plasma coater (PDC210; Yamato). Finally, the microchannels were hydrophilized using a water-soluble polymer (lipidure CR1705; NOF). The lipidure was diluted 50 times with ethanol and introduced into the microchannels with a syringe or by decompression treatment. After several minutes, the microchannels were dried using a syringe. Observation of nanotrain movement in a microchannel The 20 wt% dextran (molecular weight=100,000–200,000; Polysciences) was dissolved in the HEPES buffer (pH 7.3), and it was introduced into the microchannels with a syringe or by decompression treatment. Then, the dextran solution in the start position reservoir was replaced by the CNT–liposome nanotrain solution (ca. 20 μl). The platinum electrodes (diameter: 600 μm; Nilaco) were placed in both start and goal positions, and a voltage (50–400 V) was applied to the microchannel using a high-voltage-power-supply system (HVS448; LabSmith). The nanotrain’s movement in the microchannel was observed by fluorescence microscopy (IX70; Olympus) with a colour CCD video camera (VB-7010; Keyence). The speed of the nanotrains was analysed by image-analysis software (ImageJ; NIH). The switchback of the nanotrain movement was controlled by the software (sequence; Labsmith). The movement of λ phage DNA (32 mDa, 48502, bp; Toyobo) molecules in a microchannel was monitored in a manner similar to that in nanotrains. Before the experiments, the DNA solution (90 μl, 16 μg ml −1 ) was mixed with 1 × GelRed solution (10 μL) (Wako) as an intercalator. Laser experiments The directional molecular transport, the temperature distribution in the microchannel and the artificial molecular-signalling experiments using the laser-irradiation set-up were performed as follows. The general procedures for these experiments are illustrated in Figs 4a and 5a . A 1,064-nm NIR laser beam from a continuous-wave YVO 4 laser (BL106-C; Spectra Physics) (100–700 mW (10–69 mW μm −2 )) was incorporated into the fluorescence microscopy set-up (IX71; Olympus), as described previously [35] . The laser beam was focused into the moved nanotrains in a straight microchannel with the objective (magnification: X20, numerical aperture 0.4; Olympus) during the application of voltage (50–300 V). The fluorescence images before and during the laser irradiation were recorded using an EM-CCD camera. The sequential calcein release experiment was performed by manual laser ‘on’–‘off’ switching. The temperature distribution around the laser spot was determined from the fluorescence intensity distribution of Rh molecules on the liposomes. The control experiment for the temperature assay was also studied by introducing the biotin- and Rh-labelled liposome containing calcein without the CNT (1 mM) in the microchannel with a syringe. The fluorescence intensities of calcein, Rh and fluorescein were analysed by ImageJ. The artificial molecular-signalling experiment was performed by setting β-galactosidase from Escherichia coli (0.5 mg ml −1 ; Roche)/HEPES (pH 7.1) solution (ca. 20 μl) in the goal position reservoir. How to cite this article: Miyako E. et al . Carbon nanotube–liposome supramolecular nanotrains for intelligent molecular-transport systems. Nat. Commun. 3:1226 doi: 10.1038/ncomms2233 (2012).